Evolutionarily conserved intercalated disc protein Tmem65 regulates cardiac conduction and connexin 43 function Membrane proteins are crucial to heart function and development. Here we combine cationic silica-bead coating with shotgun proteomics to enrich for and identify plasma membrane-associated proteins from primary mouse neonatal and human fetal ventricular cardiomyocytes. We identify Tmem65 as a cardiac-enriched, intercalated disc protein that increases during development in both mouse and human hearts. Functional analysis of Tmem65 both in vitro using lentiviral shRNA-mediated knockdown in mouse cardiomyocytes and in vivo using morpholino-based knockdown in zebrafish show marked alterations in gap junction function and cardiac morphology. Molecular analyses suggest that Tmem65 interaction with connexin 43 (Cx43) is required for correct localization of Cx43 to the intercalated disc, since Tmem65 deletion results in marked internalization of Cx43, a shorter half-life through increased degradation, and loss of Cx43 function. Our data demonstrate that the membrane protein Tmem65 is an intercalated disc protein that interacts with and functionally regulates ventricular Cx43. Spontaneous heartbeats rely on proteins embedded in or associated with the cardiac sarcolemmal membrane. This membrane system includes an extensive transverse-tubular structure enriched in proteins involved in excitation–contraction coupling and specialized regions abundant in lipid rafts and caveolae required for transport and signalling. Membrane proteins in these regions act as signalling receptors, enzymes, transporters, cell–cell adhesion anchors and cell–cell signal propagators [1] . Electrical current propagation throughout the heart is mediated through precisely regulated ion movements coordinated by various cell surface and gap junction proteins [2] , [3] . A clear understanding of all of these proteins is crucial, especially when disturbances in conduction from malfunctioning membrane channels lead to cardiac arrhythmias [3] . Here we use a systematic proteomics discovery strategy to identify plasma membrane proteins from human and cultured mouse ventricular cardiomyocytes. Obtained data were systematically integrated with available microarray tissue expression profiles and phenotype ontology information ( http://www.informatics.jax.org ) to identify previously uncharacterized, cardiac-enriched membrane proteins. As a result of these analyses, we uncover Tmem65, a novel evolutionarily conserved intercalated disc protein (ICD) that interacts with connexin 43 (Cx43), the major gap junction protein in the heart. We show that both in vivo and in vitro knockdown cause dysregulation and internalization of Cx43, a mechanism common to cardiac arrhythmias. Surfaceome analysis uncovers Tmem65 In-depth studies of membrane proteins have proven to be difficult because of their low abundance and hydrophobicity [1] , [4] . However, recent advances in proteomic technologies make it possible to investigate proteins in this cell compartment, including previously unannotated membrane proteins, to an impressive depth [4] , [5] , [6] , [7] , [8] , [9] . In this study, we applied colloidal silica-bead coating [10] to enrich for conserved cell-surface-associated proteins in mouse neonatal and human fetal ventricular cardiomyocytes. We isolated a membrane-depleted homogenate (H) and a membrane-enriched pellet (P) fraction, and both sets were subjected to MudPIT (Multidimensional Protein Identification Technology) [11] analysis, database searching and statistical filtering on the peptide and protein levels (<1% false discovery rate (FDR)), followed by relative quantification based on spectral counts ( Fig. 1a ). 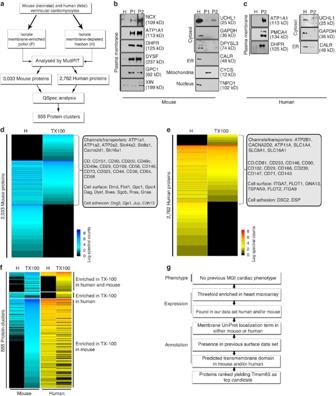Figure 1: Enrichment of cell-surface-associated proteins. (a) Schematic of the work flow that resulted in the identification of 555 membrane-enriched proteins. (b) Immunoblot analysis of mouse homogenate (H), crude pellet (P1) and purified final pellet (P2) showing enrichment of cell-surface-associated membrane proteins as monitored by: the Na+/K+ATPase (ATP1A1), Na+/Ca+exchanger (NCX), dihydropyridine receptor (DHPR), dysferlin (DYSF), glypican-1 (GPC1) and cardiomyopathy-associated protein 1 (Xin repeat-containing protein 1, XIN1). Cytoplasmic proteins: ubiquitin carboxyl-terminal esterase L1 (UCHL1) and glyceraldehyde-3-phosphate dehydrogenase (GAPDH) and dihydropyrimidinase-like 3 (DPYSL3), endoplasmic reticulum; calreticulin (CALR), mitochondria; cytochromec(CYCS) and nuclear protein; transportin-1 (TNPO1). (c) Immunoblot analysis of human homogenate (H) and final pellet (P2). Enrichment monitored by:ATP1A1, plasma membrane calcium ATPase type 4 (PMCA4) andDHPRand the depletion of known cytosolic (UCHL1,GAPDH) and ER (CALR) proteins. (d) Heatmap representation of mouse and (e) human proteins in H and P fractions with insert showing examples of identified over-represented cell-surface-associated proteins. (f) Heatmap representation of Qspec enriched 555 orthologue protein clusters based on spectral counts. (g) Schematic of the ranking of the 555 protein clusters. 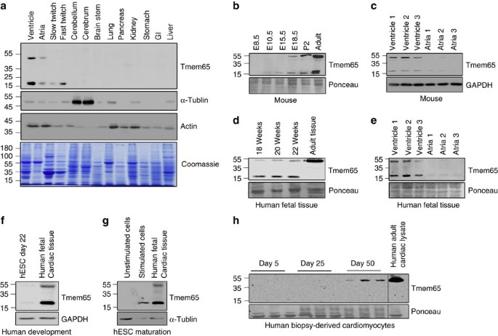Figure 2: Characterization of Tmem65 expression in mouse and human tissue. (a) Immunoblot analysis of 13 different mouse tissues probed for Tmem65 expression and loading controls α-tubulin, actin and Coomassie blue staining. (b) Immunoblots of Tmem65 in mouse embryo and postnatal cardiac tissues. (c) Immunoblots of Tmem65 in adult mouse ventricle and atria tissue. (d) Immunoblot analysis of Tmem65 in fetal ventricle tissue at different gestational ages and in human adult ventricle explant tissue. (e) Immunoblot analysis in human fetal ventricle and atria. (f) Immunoblot analysis of Tmem65 in hESC-CM on day 22 (T22) and human fetal heart tissue. (g) Immunoblot analysis of Tmem65 in unstimulated hESC-CM (T22), mechanical stretch-stimulated hESC-CM and human fetal heart tissue. (h) Immunoblot analysis ofin vitrohuman cardiosphere-derived cardiomyocytes in culture up to 50 days. Analyses of three biological repeats resulted in the identification of a final set of 3,033 mouse ( Supplementary Table 1 ) and 2,762 human proteins ( Supplementary Table 2 ). Enrichment of cell-surface-associated proteins was confirmed using western blotting analysis of known subcellular markers in both the H and P fractions ( Fig. 1b,c ). Heatmap schematics shown in Fig. 1d,e depict separation of all identified proteins into the indicated fractions, where a variety of cell-surface-associated proteins are highlighted. Comparative proteomics using the QSpec analysis [12] identified 555 differentially enriched orthologue protein clusters in the membrane-enriched versus the membrane-depleted fraction ( Fig. 1f and Supplementary Tables 3 and 4 ). To identify previously uncharacterized cell-surface-associated proteins, we applied a ranking strategy to all 555 orthologues and prioritized proteins with no previous links to cardiac function on the basis of phenotype ontology ( http://www.informatics.jax.org ) and cardiac enrichment on the basis of threefold upregulation in cardiac tissue, using publicly available microarrays [13] . This approach identified Tmem65 as our top candidate ( Fig. 1g ). Figure 1: Enrichment of cell-surface-associated proteins. ( a ) Schematic of the work flow that resulted in the identification of 555 membrane-enriched proteins. ( b ) Immunoblot analysis of mouse homogenate (H), crude pellet (P1) and purified final pellet (P2) showing enrichment of cell-surface-associated membrane proteins as monitored by: the Na + /K + ATPase ( ATP1A1 ), Na + /Ca + exchanger ( NCX ), dihydropyridine receptor ( DHPR ), dysferlin ( DYSF ), glypican-1 ( GPC1 ) and cardiomyopathy-associated protein 1 (Xin repeat-containing protein 1, XIN1). Cytoplasmic proteins: ubiquitin carboxyl-terminal esterase L1 ( UCHL1 ) and glyceraldehyde-3-phosphate dehydrogenase ( GAPDH ) and dihydropyrimidinase-like 3 ( DPYSL3 ), endoplasmic reticulum; calreticulin ( CALR ), mitochondria; cytochrome c ( CYCS ) and nuclear protein; transportin-1 ( TNPO1 ). ( c ) Immunoblot analysis of human homogenate (H) and final pellet (P2). Enrichment monitored by: ATP1A1 , plasma membrane calcium ATPase type 4 ( PMCA4 ) and DHPR and the depletion of known cytosolic ( UCHL1 , GAPDH ) and ER ( CALR ) proteins. ( d ) Heatmap representation of mouse and ( e ) human proteins in H and P fractions with insert showing examples of identified over-represented cell-surface-associated proteins. ( f ) Heatmap representation of Qspec enriched 555 orthologue protein clusters based on spectral counts. ( g ) Schematic of the ranking of the 555 protein clusters. Full size image To confirm cardiac enrichment, we characterized Tmem65 expression in different mouse organs using immunoblot (IB) analysis and demonstrated its predominant expression in cardiac tissue, with enrichment in the ventricle ( Fig. 2a ). Antibody specificity was confirmed by blocking with purified 6xHis-tagged Tmem65 ( Supplementary Fig. 1a ). These data validate Tmem65 as a novel cardiac-enriched protein. Figure 2: Characterization of Tmem65 expression in mouse and human tissue. ( a ) Immunoblot analysis of 13 different mouse tissues probed for Tmem65 expression and loading controls α-tubulin, actin and Coomassie blue staining. ( b ) Immunoblots of Tmem65 in mouse embryo and postnatal cardiac tissues. ( c ) Immunoblots of Tmem65 in adult mouse ventricle and atria tissue. ( d ) Immunoblot analysis of Tmem65 in fetal ventricle tissue at different gestational ages and in human adult ventricle explant tissue. ( e ) Immunoblot analysis in human fetal ventricle and atria. ( f ) Immunoblot analysis of Tmem65 in hESC-CM on day 22 (T22) and human fetal heart tissue. ( g ) Immunoblot analysis of Tmem65 in unstimulated hESC-CM (T22), mechanical stretch-stimulated hESC-CM and human fetal heart tissue. ( h ) Immunoblot analysis of in vitro human cardiosphere-derived cardiomyocytes in culture up to 50 days. Full size image Tmem65 is a marker of cardiomyocyte development To determine expression during development, we analysed mouse cardiac tissue from time-staged embryos and showed only low levels of Tmem65 expression between embryonic day 8.5 (E8.5) and day 15.5 (E15.5; Fig. 2b ). IB analysis indicated that expression levels increased progressively after birth, with the highest levels being seen in adults ( Fig. 2b ). An apparent dimer was detectable in later stages of heart development (P2 to adult); however, we did not detect this dimer in any other tissue types ( Fig. 2a ) or in the earliest stages of embryonic development analysed. These data suggest a possibly unique function for the dimer in the developed heart. The dimer was stable to heat even in SDS [14] , [15] , but was monomerized by heating the adult cardiac lysate in 6M urea [14] ( Supplementary Fig. 1b ). Sequence analysis identified a conserved glycine zipper motif GxxxGxxxG, known to promote homo-oligomerization [16] , [17] , located in the third predicted transmembrane region. Disulphide bonds were predicted using DIpro [18] ( http://scratch.proteomics.ics.uci.edu ), which would promote stabilization of the dimer. Truncation of Tmem65 at the glycine zipper leading to deletion of the predicted third membrane domain led to dissociation of the dimer ( Supplementary Fig. 1c ). Analysis of the expression patterns of this developmentally regulated marker in isolated ventricular and atrial samples revealed that Tmem65 is predominantly expressed in ventricular tissue ( Fig. 2c ). Two additional antibodies confirmed the presence of both monomer and dimer, and their signals were blocked when the antibodies were pre-incubated with 6xHis-Tmem65 protein overexpressed in HEK293 cells ( Supplementary Fig. 1d,e ). We performed western blot analysis of human fetal tissue between ages 18 and 22 weeks and human adult explants. Figure 2d shows the presence of the Tmem65 protein in human fetal tissues together with a >20-fold increase during human development. Analysis of differential expression between human ventricle and atrial tissue using western blot analysis confirmed our observations made in mouse tissue and showed significant differential expression between human fetal ventricle and atria ( Fig. 2e ). Generation of cardiovascular cells from human and mouse pluripotent stem cells provides a powerful model system for investigation of all aspects of cardiovascular biology. A great effort is currently underway to promote the maturation of embryo-derived stem cells by a multitude of methods, including manipulation of growth factors [19] , electrical stimulation [20] and mechanical stretching [21] . To date, monitoring the developmental stages of human embryonic stem cell (hESC)-derived cardiomyocytes (hESC-CM) has been dependent on gene expression levels and morphological changes [22] . We found higher levels of the Tmem65 protein in the fetal cells compared with the hESC-CM using IB analysis ( Fig. 2f ) and an increase in gene expression using quantitative PCR as the hESC-CM matured in culture ( Supplementary Fig. 1f ). As in the mouse, the Tmem65 dimer was present only in fetal tissue. Immature hESC-CM showed virtually no expression of Tmem65. Next, we stimulated the hESC-CM by mechanical stretching to induce maturation [23] and showed a >20-fold upregulation in Tmem65 protein levels as a result of mechanical stimulation ( Fig. 2g ). Further evidence that Tmem65 is a possible marker of mature human cardiomyocytes was obtained by the analysis of in vitro human cardiac cells derived from explants (Promocell), which showed an increase in expression from day 5 to day 50 ( Fig. 2h ) that coincides with the expression of genetic markers of maturation [24] . Thus, Tmem65 is a potentially promising marker, which could be used to monitor maturation of both mouse and human ventricular cardiomyocytes. Tmem65 is a novel ICD Immunofluorescence (IF) analysis of Tmem65 in adult mouse ventricle tissue ( Fig. 3a ; top panel) and dissociated primary adult mouse cardiomyocytes ( Fig. 3a ; bottom panel) showed its localization to be the ICD of the plasma membrane. ICD staining was further confirmed by immunogold labelling of ultrathin cryosections of mouse ventricle tissue using Tmem65 antibodies, which demonstrated intense labelling along the plasma membranes associated with the ICD, while immunogold staining using a gold-conjugated secondary antibody alone showed no gold particle labelling ( Fig. 3b and Supplementary Fig. 2 ). To examine Tmem65 expression in human tissue, we queried cardiac staining in the Human Protein Atlas database ( http://www.proteinatlas.org ) [25] and confirmed localization at the ICD in human ventricular tissue ( Fig. 3c ). These data validate Tmem65 as a cardiac-enriched membrane protein localized in the ICD. 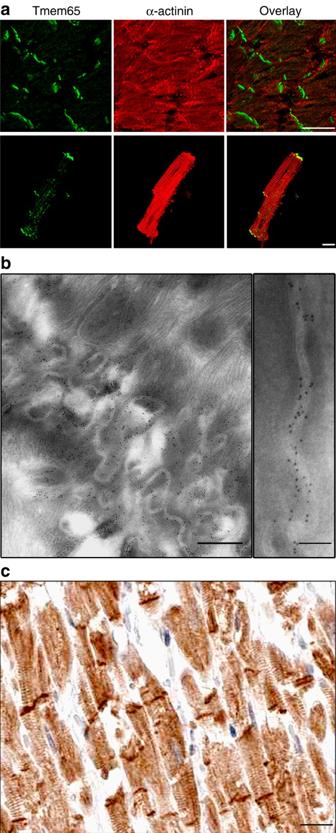Figure 3: Tmem65 localization in the intercalated disc. (a) Immunofluorescence images of mouse adult ventricle tissue sections (top panel) and isolated mouse adult cardiomyocytes with Tmem65 co-stained with cardiac sarcomeric α-actinin (bottom panel). Scale bars, 20 μm. (b) Electron micrograph of Tmem65 immunogold labelled in mouse ventricle tissue. Gold particles are confined to the ICD. Gold particles are associated with the plasma membrane from both cardiac myocytes (also seeSupplementary Fig. 2). Scale bar, left panel 500 nm; right panel, 100 nm. (c) Tmem65 staining in human cardiac tissue queried in the Human Protein Atlas database (http://www.proteinatlas.org). Scale bar, 25 μm. Figure 3: Tmem65 localization in the intercalated disc. ( a ) Immunofluorescence images of mouse adult ventricle tissue sections (top panel) and isolated mouse adult cardiomyocytes with Tmem65 co-stained with cardiac sarcomeric α-actinin (bottom panel). Scale bars, 20 μm. ( b ) Electron micrograph of Tmem65 immunogold labelled in mouse ventricle tissue. Gold particles are confined to the ICD. Gold particles are associated with the plasma membrane from both cardiac myocytes (also see Supplementary Fig. 2 ). Scale bar, left panel 500 nm; right panel, 100 nm. ( c ) Tmem65 staining in human cardiac tissue queried in the Human Protein Atlas database ( http://www.proteinatlas.org ). Scale bar, 25 μm. Full size image Tmem65 is a highly conserved Type II transmembrane protein Tmem65 is a highly conserved multipass membrane protein with no previous link to cardiac biology or function. Amino-acid sequence analysis showed 92% homology between mouse and human orthologues, 57% between mouse and zebrafish and 33% between mouse and Caenorhabditis elegans ( C. elegans ) . In silico analyses also demonstrated that Tmem65 orthologues are part of a superfamily containing a conserved DUF2453 domain of unknown function. These data suggest an essential, evolutionarily conserved function. The majority of sequence divergence occurs in exon 1, while exons 2–6 have the greatest degree of conservation from C. elegans to humans ( Fig. 4a ). Phylogenetic analysis further demonstrated clustering of mammalian taxa such as human, mouse, primates and rodents ( Supplementary Fig. 3 ). 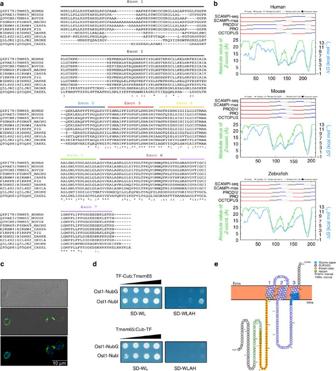Figure 4: Tmem65 sequence alignment and topology. (a) Sequence alignment shows that Tmem65 is conserved throughout multiple species and that majority of divergence occurs in exon 1. (b) Prediction of mouse, human and zebrafish Tmem65 structure using TOPCON (http://topcons.cbr.su.se). (c) Fluorescence microscopy images of Tmem65-LexA-VP16-tagged construct successfully localized to the yeast plasma membrane. Figure shows differential interference contrast (DIC) image, an overlay of Cyan Fluorescent Protein (CFP) and DIC as well as an overlay CFP and nuclear staining with 4,6-diamidino-2-phenylindole. Scale bar, 10 μm. (d) MYTH system analysis of Tmem65 membrane topology. The N-terminal-tagged Tmem65 construct (TF-Cub::Tmem65) is exposed to the cytoplasm and it allows ubiquitin (Ub) reconstitution with a cytoplasmic prey (Ost1::NubI) to activate reporter genes, but not with a mutant prey Ost1::NubG. The C terminus of Tmem65 is extracellular and the C terminally tagged Tmem65 construct (Tmem65::Cub-TF) does not interact with either the prey. SD-WL is synthetic defined (SD) yeast media that lack tryptophan (W) and leucine (L) and select for cells that contain both bait and prey plasmids. SD-WLAH is synthetic defined (SD) yeast media that lack tryptophan (W), leucine (L), adenine (A) and histidine (H), and select for cells in which bait and prey are interacting. (e) Membrane topology model generated by Protter70for Tmem65 combining predicted and MYTH assay-generated data. Selected Tmem65 domains and peptide sequences used for commercial Tmem65 antibody generation (Human Protein Atlas, Abcam) are indicated. Figure 4: Tmem65 sequence alignment and topology. ( a ) Sequence alignment shows that Tmem65 is conserved throughout multiple species and that majority of divergence occurs in exon 1. ( b ) Prediction of mouse, human and zebrafish Tmem65 structure using TOPCON ( http://topcons.cbr.su.se ). ( c ) Fluorescence microscopy images of Tmem65-LexA-VP16-tagged construct successfully localized to the yeast plasma membrane. Figure shows differential interference contrast (DIC) image, an overlay of Cyan Fluorescent Protein (CFP) and DIC as well as an overlay CFP and nuclear staining with 4,6-diamidino-2-phenylindole. Scale bar, 10 μm. ( d ) MYTH system analysis of Tmem65 membrane topology. The N-terminal-tagged Tmem65 construct (TF-Cub::Tmem65) is exposed to the cytoplasm and it allows ubiquitin (Ub) reconstitution with a cytoplasmic prey (Ost1::NubI) to activate reporter genes, but not with a mutant prey Ost1::NubG. The C terminus of Tmem65 is extracellular and the C terminally tagged Tmem65 construct (Tmem65::Cub-TF) does not interact with either the prey. SD-WL is synthetic defined (SD) yeast media that lack tryptophan (W) and leucine (L) and select for cells that contain both bait and prey plasmids. SD-WLAH is synthetic defined (SD) yeast media that lack tryptophan (W), leucine (L), adenine (A) and histidine (H), and select for cells in which bait and prey are interacting. ( e ) Membrane topology model generated by Protter [70] for Tmem65 combining predicted and MYTH assay-generated data. Selected Tmem65 domains and peptide sequences used for commercial Tmem65 antibody generation (Human Protein Atlas, Abcam) are indicated. Full size image To determine membrane topology we used the multi-algorithm prediction tools available at the TOPCON website ( http://topcons.cbr.su.se ). All five prediction algorithms encompassed within this tool determined that the N terminus was cytoplasmic for both mouse and human Tmem65; however, three transmembrane helices were predicted at the C terminus in some programmes and four in others ( Fig. 4b ). The prediction models suggested an overall consistent three transmembrane helix membrane topology for the zebrafish orthologue ( Fig. 4b ). To determine the actual membrane topology of human Tmem65, we employed a membrane yeast two-hybrid (MYTH) system, as previously described ( Fig. 4c,d ) [26] , [27] , [28] . To determine protein topography, both N-terminal (TF-Cub-Tmem65) and C-terminal (Tmem65-Cub-TF) ‘bait’ Tmem65 proteins were tested for protein–protein interactions (PPIs) in the presence of a non-interacting yeast integral membrane protein Ost1p (ref. 27 ) fused to either NubI (Ost1–NubI) or NubG (Ost1–NubG). The Ost1–NubI control ‘prey’ construct is designed to activate the yeast reporter system, irrespective of a PPI because of the high affinity with which NubI associated with Cub to form active ubiquitin, but only if the Cub domain of the corresponding ‘bait’ protein is localized in the cytosol. Activation of the reporter system was measured as growth on media lacking histidine and adenine in the presence of X-gal. This NubG/I assay verified that the N terminally tagged Tmem65 construct, but not the C terminally tagged ‘bait’, interacted with the Ost1–NubI control prey ( Fig. 4d ), indicating that the N terminus was intracellular and the C terminus of Tmem65 was extracellular. We propose that human Tmem65 contains a cytoplasmic N terminus, an extracellular C terminus and three transmembrane sequences ( Fig. 4e ). Tmem65 is essential for cardiac function in zebrafish To assess Tmem65 function in vivo , we took advantage of the rapid development of zebrafish (Danio rerio) , in which expression of Tmem65 was first evident by western blotting 3 days post fertilization (dpf; Fig. 5a ). IF showed Tmem65 expression to be restricted to the zebrafish heart ( Fig. 5b ), consistent with our observations in mouse. To assess the role of Tmem65 in cardiac function, we injected an antisense tmem65 morpholino (tmem65-MO) in zebrafish embryos, and western blots confirmed an effective knockdown of Tmem65 expression ( Fig. 5c ). Loss of Tmem65 was associated with pericardial oedema and altered cardiac morphology at 4 dpf in Tmem65-MO morphant embryos and severity increased as embryos aged, when compared with control fish ( Fig. 5d and Supplementary Fig. 4a ). Tmem65-MO morphants were not viable by 7 dpf, suggesting an essential function of Tmem65 in early stages of cardiac development ( Fig. 5d ). Detailed analysis of zebrafish hearts showed abnormal cardiac looping in the morphants when compared with control fish ( Fig. 5e–g and Supplementary Fig. 4b ). A significant decline in heart beat rates was also monitored in Tmem65-MO morphants after 4.5 dpf ( Supplementary Fig. 5a ) and continued decreasing at 5 and 6 dpf ( Supplementary Movie 1 for a control and Supplementary Movie 2 for 6 dpf Tmem65-MO morphant). Whole-tissue Ca 2+ transients in fish ventricles showed a significant reduction in Ca 2+ amplitude in Tmem65-MO morphants between 4 and 6 dpf. 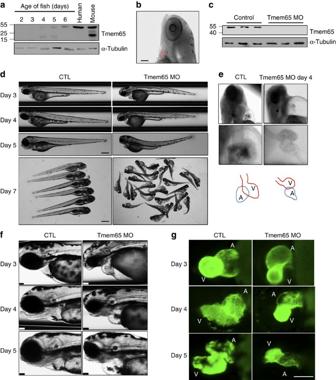Figure 5:In vivophenotype analysis of Tmem65 knockdown in zebrafish. (a) Immunoblot analysis of Tmem65 in wild-type zebrafish(Danio rerio)at developmental time points shows expression starting at 3 dpf. (b) Immunofluorescence of Tmem65 in wild type. Scale bar, 25 μm. (c) Immunoblot analysis of day 4 morphant-mediated Tmem65 knockdown in zebrafish. (d) Analysis of control (CTL) and Tmem65 morphant fish from 3 to 7 dpf. Scale bar, 100 μm. (e) CTL and Tmem65 morphant fish at 4 dpf at higher magnification of the chest. Scale bar, 20 μm. The heart chambers were highlighted in outline tracings. (f) Brightfield imaging of 3–5 dpf CTL and Tmem65 morphant fish. Pericardial oedema is evident at 3 dpf in the Tmem65 morphants. Scale bar, 20 μm. (g) GFP imaging of the hearts show cardiac looping defects as early as 3 dpf in the Tmem65 morphants. Scale bar, 10 μm. Interestingly, no significant changes were detected in the atrial Ca 2+ transients of Tmem65-MO morphants ( Supplementary Fig 5b ). These data are consistent with the low protein expression seen in the atria and highlight a potentially essential role of Tmem65 in the ventricle in vivo. Altogether, Tmem65 is a cardiac-specific protein that plays an essential role during cardiac development. Loss of Tmem65 is associated with aberrant Ca 2+ transients and reduced cardiac contractility. Figure 5: In vivo phenotype analysis of Tmem65 knockdown in zebrafish. ( a ) Immunoblot analysis of Tmem65 in wild-type zebrafish (Danio rerio) at developmental time points shows expression starting at 3 dpf. ( b ) Immunofluorescence of Tmem65 in wild type. Scale bar, 25 μm. ( c ) Immunoblot analysis of day 4 morphant-mediated Tmem65 knockdown in zebrafish. ( d ) Analysis of control (CTL) and Tmem65 morphant fish from 3 to 7 dpf. Scale bar, 100 μm. ( e ) CTL and Tmem65 morphant fish at 4 dpf at higher magnification of the chest. Scale bar, 20 μm. The heart chambers were highlighted in outline tracings. ( f ) Brightfield imaging of 3–5 dpf CTL and Tmem65 morphant fish. Pericardial oedema is evident at 3 dpf in the Tmem65 morphants. Scale bar, 20 μm. ( g ) GFP imaging of the hearts show cardiac looping defects as early as 3 dpf in the Tmem65 morphants. Scale bar, 10 μm. Full size image Tmem65 is a novel regulator of the gap junction Since we identified Tmem65 localization to the ICD, we next carried out more systematic analyses of its localization and possible binding partners. Briefly, we performed IF microscopy with the ICD proteins Cx43, N-cadherin (NCAD) and desmoplakin (DSP) and calculated Pearson coefficients for colocalization. A Pearson coefficient of >0.5 is considered statistically significant and represents colocalization of the proteins of interest [29] . The two-dimensional ( Fig. 6a ; left panel) and three-dimensional ( Fig. 6a ; right panel) fluorescence images demonstrated that Tmem65 and Cx43 colocalized with a statistically significant Pearson coefficient of 0.64±0.07, similar to the Pearson coefficient for Tmem65 and NCAD of 0.62±0.03. However, Tmem65 and DSP showed no significant colocalization, since the Pearson coefficient was only 0.37±0.07. To further assess the colocalization findings, we performed immunoprecipitation assays with adult mouse cardiac lysates together with anti-Cx43, anti-NCAD and anti-DSP antibodies. IB analysis showed that the Tmem65 monomer and dimer co-immunoprecipitated with Cx43, although significant enrichment was observed in the dimer, compared with levels seen in the input cardiac lysate. Low levels of Tmem65 dimer were detected in the immunoprecipitation with anti-DSP, and no enrichment was seen in the immunoprecipitation with anti-NCAD. Background levels were determined using protein A/G beads alone ( Fig. 6b ). All three antibodies were able to immunoprecipitate their respective antigens from cardiac lysate, indicating their apparent suitability for co-immunoprecipitation ( Fig. 6b ; right panels). 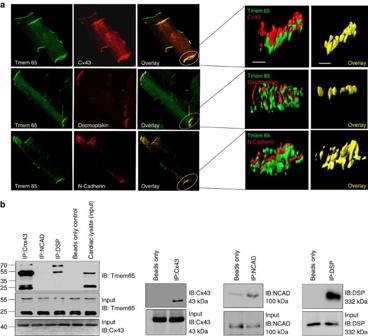Figure 6: Membrane localization of Tmem65 (a) Immunofluorescence of adult mouse cardiomyocytes shows colocalization of the three ICD proteins Cx43, DSP and NCAD with Tmem65 at the ICD. Right panel, three-dimensional rendering of colocalization. Scale bar, 4 μm. (b) Immunoprecipitation of known intercalated disc proteins Cx43, NCAD, DSP from mouse heart lysates. IgG beads alone were used as controls. Each antibody demonstrated the ability to immunoprecipitate itself from cardiac lysate (right panels). Figure 6: Membrane localization of Tmem65 ( a ) Immunofluorescence of adult mouse cardiomyocytes shows colocalization of the three ICD proteins Cx43, DSP and NCAD with Tmem65 at the ICD. Right panel, three-dimensional rendering of colocalization. Scale bar, 4 μm. ( b ) Immunoprecipitation of known intercalated disc proteins Cx43, NCAD, DSP from mouse heart lysates. IgG beads alone were used as controls. Each antibody demonstrated the ability to immunoprecipitate itself from cardiac lysate (right panels). Full size image Cx43 function is strongly regulated by its localization and protein stability [30] , [31] , [32] . Therefore, we examined Cx43 levels and localization in control and Tmem65 knockdown cells. Silencing of Tmem65 through transduction with LentiVectors expressing short hairpin RNA (shRNA) for Tmem65 in mouse neonatal cardiomyocytes (mNCMs) was confirmed by western blotting ( Fig. 7a ). Since internalization of Cx43 is the first step in its degradation [33] , [34] , we performed IF analyses of control-transduced mNCMs that showed clear staining of Cx43 at the ICD, whereas Tmem65-silenced cells showed less membrane staining and internalization of Cx43 ( Fig. 7b ). This was confirmed by sucrose density organelle fractionation [35] , which showed Cx43 in the Tmem65 knockdown neonatal cardiomyocytes to be reduced in amount and to shift from a more dense membrane fraction to a less dense cytosolic fraction ( Fig. 7c ). 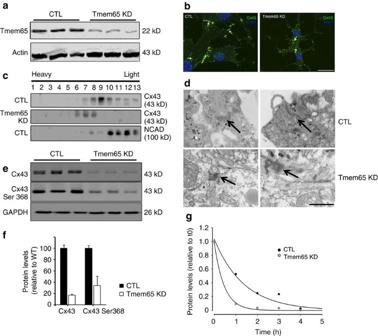Figure 7: Tmem65 knockdown affects Cx43 levels. (a) Immunoblots of Tmem65 knockdown using shRNA in mNCM. (b) Immunofluorescence of wild-type and Tmem65 knockdown neonatal mouse cardiomyocytes showing internalization of Cx43. Scale bar, 10 μm. (c) Immunoblot of Cx43 in wild type and knockdown neonatal mouse cardiomyocytes analysed using continuous sucrose density gradient. (d) Electron micrographs of neonatal cardiomyoctes transfected with a scrambled vector or Tmem65 KD shRNAs. Arrows highlight the intercalated discs between two adjacent myocytes. Scale bar, 500 nm. (e) Immunoblot analysis of Cx43 and phospho-Cx43Ser386 levels in wild-type and knockdown neonatal mouse cardiomyocytes. (f) Quantitative analysis of immunoblots. Mean±s.e.m.,n=3. (g) Half-life of Cx43 using [35S]-methionine and [35S]-cysteine to carry out a pulse chase experiment in wild-type and Tmem65 knockdown neonatal mouse cardiomyocytes (data obtained from four pooled 35-mm culture plates). Figure 7: Tmem65 knockdown affects Cx43 levels. ( a ) Immunoblots of Tmem65 knockdown using shRNA in mNCM. ( b ) Immunofluorescence of wild-type and Tmem65 knockdown neonatal mouse cardiomyocytes showing internalization of Cx43. Scale bar, 10 μm. ( c ) Immunoblot of Cx43 in wild type and knockdown neonatal mouse cardiomyocytes analysed using continuous sucrose density gradient. ( d ) Electron micrographs of neonatal cardiomyoctes transfected with a scrambled vector or Tmem65 KD shRNAs. Arrows highlight the intercalated discs between two adjacent myocytes. Scale bar, 500 nm. ( e ) Immunoblot analysis of Cx43 and phospho-Cx43Ser386 levels in wild-type and knockdown neonatal mouse cardiomyocytes. ( f ) Quantitative analysis of immunoblots. Mean±s.e.m., n =3. ( g ) Half-life of Cx43 using [ 35 S]-methionine and [ 35 S]-cysteine to carry out a pulse chase experiment in wild-type and Tmem65 knockdown neonatal mouse cardiomyocytes (data obtained from four pooled 35-mm culture plates). Full size image Transmission electron microscopy of ultrathin sections of cultured mNCMs showed altered cellular junctions in Tmem65 knockdown cells compared with the symmetrical cellular membranes and connections in the scrambled control cells ( Fig. 7d ). These data suggest that Tmem65 knockdown could affect cellular communication by either Cx43 internalization and/or structural alterations of cellular junctions. Localization of Cx43 has previously been monitored by changes in Cx43 phosphorylation at Ser 325, Ser 328, Ser 330 and Ser 368 (ref. 36 ), although commercial antibodies were only found for Ser 368. Since we observed an ∼ 83% reduction in the total Cx43 protein levels in Tmem65 knockdown (KD) mNCM ( Fig. 7e ), we compared the levels of Ser 368 phosphorylation as a percentage of the total Cx43. We found that total Cx43 protein levels were reduced by ∼ 83%, and the phosphorylated levels reduced by 67%. The resulting ratio of phosphorylated:non-phosphorylated Cx43 increased by a relative approximately twofold ( Fig. 7f ). Relative increases in levels of Ser 368-phosphorylated Cx43 have previously been suggested to be involved in increased internalization and degradation of Cx43 (ref. 37 ). Consistent with these findings, we determined a significant reduction in the Cx43 half-life from 1.8 h (ref. 38 ) to 1.2 h in Tmem65 knockdown mouse cardiomyocytes by pulse chase ( Fig. 7g ). In line with these data, Tmem65 knockdown in zebrafish resulted in marked reduction of ventricular Cx43 ( Supplementary Fig. 6 ). Regulation of cardiac communication via Tmem65 Cx43 has long been known to be the principle conductor of the intercellular current in ventricular cardiomyocytes [39] , [40] . Since we identified Tmem65 as a protein that interacts with and regulates Cx43 expression/localization, we hypothesized that Tmem65 is functionally involved in regulating gap junction communication. To assay junctional conductance directly, we injected the membrane-impermeable dye 8-hydroxypyrene-1,3,6-Trisulfonic acid into one cell and monitored its transfer into adjacent cells across mNCM plated as a monolayer. These studies showed a significant reduction in the dye transferred to adjacent cells in the Tmem65 KD cultures (1.3±0.6 cells) in comparison with those injected with scrambled control shRNA (16±1.0 cells; P <0.001, Student’s t -test, n =3; Fig. 8a,b ). Taken together, these data imply that Tmem65 aids in the retention of Cx43 at the ICD and that knockdown causes internalization of Cx43, leading to impaired gap junction communication. 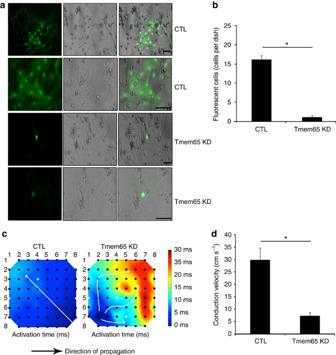Figure 8:In vitrofunctional analysis of Tmem65 knockdown in mNCM. (a) Brightfield and immunofluorescence images of junctional dye transfer assay using green Hydroxypyrene-1,3,6-Trisulfonic Acid, Trisodium Salt (HTTS) dye in lentivirally transduced myocytes using scrambled or Tmem65 KD vectors. Higher-power magnification images are shown in the second panels. Scale bar, 25 μm. (b) Quantification of junctional dye transfer assays in scram type and Tmem65 knockdown in mNCM. Asterisks (*) denote a significant decrease (mean±s.e.m.,P≤0.001, Student’st-test). (c) Representative trace of optical mapping performed using di-4-ANEPPS in scram and Tmem65 KD mNCM. (d) Electrical conduction velocities were determined using microelectrode array (MEA) plates. *indicates significant difference between scrambled and Tmem65 knockdown (mean±s.e.m., Student’st-test,P<0.01;n=5 experiments). Figure 8: In vitro functional analysis of Tmem65 knockdown in mNCM. ( a ) Brightfield and immunofluorescence images of junctional dye transfer assay using green Hydroxypyrene-1,3,6-Trisulfonic Acid, Trisodium Salt (HTTS) dye in lentivirally transduced myocytes using scrambled or Tmem65 KD vectors. Higher-power magnification images are shown in the second panels. Scale bar, 25 μm. ( b ) Quantification of junctional dye transfer assays in scram type and Tmem65 knockdown in mNCM. Asterisks (*) denote a significant decrease (mean±s.e.m., P ≤0.001, Student’s t -test). ( c ) Representative trace of optical mapping performed using di-4-ANEPPS in scram and Tmem65 KD mNCM. ( d ) Electrical conduction velocities were determined using microelectrode array (MEA) plates. *indicates significant difference between scrambled and Tmem65 knockdown (mean±s.e.m., Student’s t -test, P <0.01; n =5 experiments). Full size image Electrical defects between myocytes, as measured by a reduction in electrical conductance velocity, has been linked previously to the internalization and degradation of Cx43 (ref. 41 ). We assessed electrical conduction in the scrambled control and Tmem65 shRNA cardiomyocytes using optical mapping with the electrically sensitive imaging dye, di-4-ANEPPS, and by direct electrical conduction recordings using microelectrode arrays. Optical mapping experiments showed maximum activation rates in control cultures to be <10 ms, whereas cultures with Tmem65 KD had a discordance of synchronicity in the field of view, along with activation times in the range of 15–>30 ms ( Fig. 8c ). More precise electrical conductance measurements were performed using microelectrode array plates and calculating the electrical conduction velocities. In these studies, and consistent with the optical mapping, observations over multiple electrodes suggested a discordance of synchronicity of electrical conductance in the Tmem65 knockdown cells that resulted in electrical conduction velocities of 7.3±1.2 cm s −1 in the Tmem65 KD cultures, compared with 26.3±4.4 cm s −1 in the scrambled control cultures ( Fig. 8d , P <0.05, Student’s t -test, n =5). Taken together, these data imply that Tmem65 aids in the retention of Cx43 at the ICD and that knockdown causes internalization of Cx43, leading to reduced conductance velocity. Crucial to the understanding of human disease mechanisms is the understanding of normal physiology, which has proven to be difficult since healthy human cardiac tissue is not available. In this study we provide the first in-depth proteomic profiling of healthy human and mouse cardiomyocyte plasma membrane protein expression. Owing to the low abundance and hydrophobic nature of membrane proteins, such as Tmem65, this class of proteins has been underrepresented in proteomics studies. A comparative proteomics approach, coupled to protein ranking, identified Tmem65 as a previously uncharacterized, cell-surface-associated protein with cardiac-enriched expression. Tmem65 expression was demonstrated to be remarkably specific to ventricular cardiomyocytes. Moreover, it was developmentally regulated, and it physically interacted with the ventricular gap junction protein Cx43. Disruption of this interaction in vitro through the knockdown of Tmem65 protein expression resulted in altered cellular coupling, possibly through Cx43 mislocalization. Knockdown of the zebrafish orthologue phenocopied these results, suggesting both evolutionary conservation and a fundamental, but previously unrecognized role of Tmem65 in cardiac biology. Our data show that Tmem65 is colocalized with Cx43 in the cardiac intercalated disc, where it contributes to the localization and stability of Cx43, thereby regulating gap junction function. We also cannot rule out that Tmem65 may affect Cx43 function, and perhaps other ICD proteins, in alternative manners. Gap junctions are intercellular channels, providing a direct passage for ions and small molecules between adjacent cells, and the major communication pathway between neighbouring cells. These gap junctions are formed by Cx43, zonula occludens-1 and Xin repeat-containing protein [42] , [43] . As the main physiological function of gap junctions is to synchronize neighbouring cells electrically and/or metabolically [44] , they are the key channels that ensure rapid propagation of action potentials through the myocardium. Each gap junction channel is formed by docking of two hemichannels, called connexons. Connexons are either homo- or hetero-oligomeric proteins of up to 24 homologous connexins (Cxs). Each Cx has its own tissue distribution and each cell, with a few exceptions, expresses one or more Cxs. Cx43, Cx40, Cx45 and Cx31 are found in the cardiomyocytes of the human heart [45] , [46] . Cx43 is the major ventricular Cx responsible for gap junction coupling in ventricles. Mutations [47] , changes in expression [30] , [48] and altered post-translation modifications of Cxs [49] are the underlying mechanisms for several conditions leading to cardiac arrhythmias. Germline deletion of the Cx43 gene in mice leads to perinatal lethality due to developmental cardiac malformation [30] . In contrast, mice with cardiac-restricted inactivation of Cx43 are viable; however, they develop ventricular tachyarrhythmias leading to sudden cardiac death within 2 months [50] , [51] . Several mutations in Cx43 have previously demonstrated serious conduction abnormalities both in mouse models and in human patients [47] , [52] , [53] , [54] , [55] . Our Tmem65 knockdown results are in line with the Cx43 deletion in mouse [30] and the Cx43 deletion in the zebrafish [56] , and suggest an essential and important function for these two interacting proteins in cardiac development/function. Indeed, in all three of these cases, changes in Ca 2+ cycling, cell development and abnormal heart morphology were observed, highlighting the coordinated interactions and physiological roles of these two proteins. Furthermore, investigation of publicly available cardiac hypertrophy microarray data and protein expression in our published study of a mouse model of dilated cardiomyopathy, based on the R9C point mutation of phospholamban [57] , demonstrated decreased and coordinated expression of both Tmem65 and Cx43 ( Supplementary Fig. 7a,b ), suggesting a potential link to cardiac disease. In fact, knockdown of Tmem65 in neonatal cardiac mycocytes and in live zebrafish resulted in marked reduction in ventricular Cx43 expression, further strengthening our observation that there is correlated expression between Cx43 and Tmem65. In the context of cardiac disease, it is interesting to note that analysis of a major quantitative trait locus for heart rate (heart rate quantitative locus; hqr2; MGI:2662842) was shown to map to the chromosomal region centred on Tmem65 in the mouse [58] , further suggesting a potential role for Tmem65 as a contributor to heart rate regulation. The exact mechanistic link between these correlative observations and heart disease will require more detailed investigations in the future. Overall, our data suggest that Tmem65 is an evolutionarily conserved protein, crucial for cardiac biology, as reflected by its high sequence homology from human to C. elegans and our own data demonstrating functional conservation in human, mouse and zebrafish cardiomyocytes. Our findings provide a new paradigm of intercalated disc regulation that may translate into novel targets for potential therapeutic intervention, not only for human cardiac disease and arrhythmia, but also for a variety of human pathologies stemming from cell–cell communication dysregulation. Silica-bead extraction of cell-surface-associated proteins Plasma membrane fractions from primary neonatal cardiomyocytes were isolated using a modified cationic silica-bead plasma membrane isolation procedure [8] , [59] . Plated cardiomyocytes were first washed three times with MES-buffered saline (MBS; 25 mM 2-(N-morpholino)ethanesulfonic acid (MES), pH 6.5 and 150 mM NaCl) and then coated with 1% ice-cold silica beads for 10 min, washed three times in MBS and then incubated in 0.1% polyacrylic acid to block the free cationic groups on the silica beads. The cells were then harvested in 1 ml of sucrose/HEPES solution and were centrifuged at 1,000 g for 5 min. The homogenate was removed and labelled the ‘H’ fraction. The pellet was resuspended in 1 ml of sucrose/HEPES solution. An aliquot of this pellet at this step was removed and labelled as crude pellet (P1). The remaining P1 fraction was mixed with 50% Nycodenz solution and overlayed on a 27–40% discontinuous Nycodenz gradient and was centrifuged at 110,000 g for 1 h. The resulting pellet containing the membrane fraction bound to the silica beads (termed P2) was then eluted before mass spectrometry analysis. Plasma membrane fraction analysis (from isolated human fetal cardiomyocytes) was carried out as described for the mouse neonatal cells, but with the cells in solution and pelleted at 1,000 g after incubation with 1% silica-bead solution and each MBS wash, and later incubated in 0.1% polyacrylic acid. Homogenization and purification on the Nycodenz gradient were carried out identically to the plated mouse neonatal cells. Elution of silica-bead-bound proteins Silica beads/membrane pellicles were resuspended in NET Buffer (400 mM NaCl, 25 mM HEPES, pH 7.4, 1% Trition X-100) for 1 h at 4 °C. This was followed by centrifugation at 21,000g for 30 min at 4 °C. The supernatant was removed and precipitated in 10% trichloroacetic acid in acetone overnight at −20 °C and then centrifuged at 5,510 g at 4 °C for 20 min. The pellet was resuspended in 8 M urea and 2 mM dithiothreitol and then carboxyamidomethylated with 10 mM iodoacetamide for 1 h at 37 °C in the dark. Samples were diluted with 50 mM ammonium bicarbonate, pH 8.5 to ∼ 1.5 M urea and trypsinized overnight at 37 °C. Multidimensional protein identification technology A quaternary HPLC pump was interfaced with a Linear Trap Quadrupole (LTQ) linear ion-trap mass spectrometer (Thermo Fisher Scientific, Canada) equipped with a nanoelectrospray source (Proxeon Biosystems, Denmark). A 100-μm inner diameter-fused silica capillary (InnovaQuartz, USA) was pulled to a fine tip using a P-2000 laser puller (Sutter Instruments, Novato, Canada) and packed with ∼ 7 cm of Jupiter 4 μ Proteo 90 Å C 12 reverse phase resin (Phenomenex, USA), followed by ∼ 5 cm of Luna 5 μ 100 Å strong cation exchange resin (Phenomenex). Samples were loaded manually on separate columns using an in-house pressure vessel. As peptides eluted from the microcapillary columns, they were electrosprayed directly into the mass spectrometer (MS). A distal 2.3-kV spray voltage was applied to the microsplitter tee (Proxeon Biosystems). The MS operated in a cycle of one full-scan mass spectrum (400–1,400 m z −1 ), followed by six data-dependent MS/MS spectra at 35% normalized collision energy, which was continuously repeated throughout the entire MudPIT separation. The MS functions and the HPLC solvent gradients were controlled using the Xcalibur data system (Thermo Fisher Scientific, USA). Peptide identification and grouping Raw files were converted to m / z XML using ReAdW and searched using a locally installed version of X!TANDEM (version 2010.12.01.1) against a mouse or human UniProt database (version 2011_03, containing 16,351 mouse or 20,227 human protein sequences). To estimate and minimize our false-positive rate, the protein sequence database also contained every protein sequence in its reversed amino-acid orientation ( target-decoy strategy ) as recently described [60] . Search parameters were as follows: Parent ion Δ-mass of 4 Da, fragment mass error of 0.4 Da and complete carbaminomethyl modification of cysteine by iodoacetic acid (IAA) and a potential oxidation of cysteine. A rigorous peptide quality-control strategy was applied to effectively minimize false-positive identifications, as recently described [61] . For the presented study, we have set the value of total reverse spectra to total forward spectra to 0.5%, resulting in a low number of decoy sequences in the final output (17 reverse proteins in the mouse data and 6 reverse proteins in the human data; FDR<1%). Only fully tryptic peptides matching these criteria were accepted to generate the final list of identified proteins. We only accepted proteins identified with two unique peptides per analysed fraction (that is, H and TX-100 silica ). To minimize protein inference, we developed a database grouping scheme, and only report proteins with substantial peptide information to confirm the rules of parsimony, as recently reported [61] . Orthology mapping and Qspec analysis Since our goal was to identify conserved plasma membrane-associated proteins, we first performed orthology mapping for all identified human and mouse proteins using the MGI orthology database ( http://www.informatics.jax.org ), considering only one-to-one orthology, in a similar manner as recently reported [62] . This resulted in 2001 human–mouse one-to-one orthologues. Next, we independently performed Qspec analysis on the human and mouse orthologues to identify proteins enriched in the TX-100-eluted silica-bead fraction. Only proteins with a significant Qspec enrichment in the TX-100-eluted silica-bead fraction (FDR≤5%) in human, mouse or both species were further considered. This resulted in 555 plasma membrane-enriched orthologue proteins. Using our in-house database we performed a systematic mapping against a variety of available resources: (1) BioGPS microarray data to select cardiac-enriched transcripts; (2) a previously reported cardiac phenotype ( http://www.informatics.jax.org ); (3) a previously reported human surfaceome data set [63] ; (4) predicted transmembrane domains using TMHMM version 2 ( http://www.cbs.dtu.dk/services/TMHMM ); and (5) UniProt annotations membrane , plasma membrane , cell-surface or secreted. LentiVector production and transduction of cardiomyocytes Second-generation LentiVector-compatible clones expressing shRNAs targeting mouse TMEM65 were obtained from OpenBiosystems. We used the second-generation LentiVector system (a kind gift from Dr Jason Moffat, University of Toronto) [64] . For lentiviral production, packaging plasmid pCMV-R8.74psPAX2 (2.5 μg), envelope plasmid VSV-G/pMD2.G (0.3 μg) and the target construct plasmids in pLKO.1 (2.7 μg) were used [65] , [66] . The target vector expressed either the specific shRNAs or scrambled shRNA and was simultaneously transfected with the envelope and packaging construct into HEK-293T cells with Optimem (Invitrogen)-diluted FuGene (Roche). Following 48 h post transfection, lentivector-containing media were collected from HEK-293T cells and incubated with neonatal cardiomyocytes. Cells were incubated for up to 24 h, and the media replaced daily thereafter. After 72 h, transduced cells were incubated with DMEM/F12 media with 2% fetal bovine serum, 50 units of penicillin, 50 μg of streptomycin ml −1 , 100 μM 5-bromodeoxyuridine and 2 μg ml −1 puromycin for 48 h, for positive selection. Western blotting and IF IB analyses were performed using standard SDS–PAGE chemiluminescent procedures and antibodies used were as follows: Rabbit polyclonal to Tmem65 antibody (HPA025020, Sigma; 1:500 dilution for IB; 1:1,000 dilution for IF), rabbit polyclonal to Tmem65 antibody (ab107871, Abcam; 1:400 dilution for IB), Tmem65 (sc-87464, Santa Cruz; 1:400 dilution for IB), rabbit polyclonal to the Na + /Ca + exchanger (32881, Santa Cruz; 1:200 dilution for IB), mouse monoclonal Na + /K + ATPase (a6F, Developmental Studies Hybridoma Bank; 1:500 dilution for IB), rabbit ubiquitin carboxyl-terminal esterase L1 (U5383, Sigma; 1:2,000 dilution for IB), chicken polyclonal glyceraldehyde-3-phosphate dehydrogenase (Ab14247, Abcam; 1:1,000 dilution for IB), calreticulin (Ab2907, Abcam; 1:1,000 dilution for IB), mouse monoclonal cytochrome c (456100, Invitrogen; 1:1,000 dilution for IB), mouse monoclonal transportin-1 (ab10303, Abcam; 1:1,000 dilution for IB), mouse dysferlin (PA1-20910, Affinity Bioreagents; 1:200 dilution for IB), rabbit polyclonal glypican-1 (ab55971, Abcam; 1:500 dilution for IB), mouse dihydropyridine receptor alpha-2 (MA3-921, Affinity Bioreagents; 1:500 dilution for IB), mouse cardiomyopathy-associated 1 (611524, BD Transduction Laboratories; 1:1,000 dilution for IB), dihydropyrimidinase-like 3 protein (AB5454, Millipore; 1:2,500 dilution for IB), ryanodine receptor 2 (34C, Life Technologies; 1:2,500 dilution for IB), histidine tag (6xHis, AB18184, Abcam; 1:1,000 dilution for IB), Cx43 (AB66151, Abcam; 1:500 dilution for IB, 1:50 for IF), desmoplakin (AB16434, Abcam; 1:200 dilution for IB, 1:100 for IF), NCAD (AB18203, Abcam; 1:200 dilution for IB, 1:100 for IF), alpha-tubulin (2144, Cell Signaling; 1:1,000 for IB), actin (4967, Cell Signaling; 1:2,000 for IB), plasma membrane Ca2+ ATPase (MA3-914, Thermo Scientific; 1:1,000 for IB) and alpha actinin (MA1-22863, Fisher; 1:400 for IF). Secondary antibodies of anti-mouse IgG horse radish peroxidase (HRP) conjugate (W402B, Promega; 1:2,500 dilution) and anti-rabbit IgG HRP (W401B, Promega; 1:2,500 dilution) were used. Uncropped images for blots are provided as Supplementary Fig. 8 . Adult cardiomyocytes were dissociated from mouse ventricular tissue and stained [67] . Ventricle tissue was first washed in Hanks solution (136 mM NaCl, 4.16 mM NaHCO 3 , 0.34 mM NaH 2 PO 4 , 5.36 mM KCl, 0.44 mM KH 2 PO 4 , 5.55 mM Dextrose and 5 mM HEPES) and then isolated into approximately five pieces and incubated in Hanks solution containing 1 mg ml −1 collagenase overnight at room temperature with gentle shaking. The tissue was then transferred into dissociation solution (Hanks solution with 10 mM taurine, 0.1 mM EGTA, 10 mM butanedione monoxime (BDM), 1 mg ml −1 BSA and 1 mg ml −1 collagenase) and was rotated gently at 37 °C for 5 min. This step was repeated four times. Once dissociated, the cells were washed in PBS and then fixed for 30 min in 2% paraformaldehyde (PFA) at 4 °C. For IF, samples were blocked with 5% horse serum in permeabilization buffer (0.2% Tween-20, 0.5% Triton X-100 in PBS pH 7.0) for 30 min, and then the samples were incubated with primary antibodies in permeabilization buffer overnight at 4 °C. Samples were then washed at least three times with PBS, followed by incubation with either Alexa Fluor 488 (A11055, A21202 or A11034, Invitrogen; 1:750 dilution); Alexa Fluor 555 (A21422, A21429, Invitrogen; 1:750 dilution) or Alexa Fluor 633 (A21052, A21071; Invitrogen; 1:750 dilution). Images were collected by using a Leica DM IRBE inverted microscope equipped with a Leica TCS SP laser scanning confocal system or a Zeiss 200M fluorescent microscope. For optical mapping experiments, cultures were incubated with the voltage-sensitive dye, Di-4-ANEPPS, 5 μM; Invitrogen) for 20 min at 37 °C. Dye fluorescence was recorded on a Zeiss spinning disk equipped with a high-speed camera (Rolera). Electron microscopy Hearts were fixed in 4% PFA containing 0.1% glutaraldehyde in 0.1 M phosphate buffer pH 7.4. Tissues were then sliced into 1-mm 3 pieces, which were cryoprotected in 2.3 M sucrose. Individual pieces were then mounted on aluminium cryomicrotomy pins, frozen in liquid N2 and sections of ∼ 80 nm prepared using a cryo-ultramicrotome at −120 °C (Leica Ultracut R, Leica Microsystems, Willowdale, Canada). The sections were then transferred to formvar-coated nickel grids in a loop of molten sucrose. The grids were then treated with PBS containing 1% glycine and 0.5% BSA, rinsed in PBS BSA and incubated in Tmem65 (Sigma) antibody at a dilution of 1:10 for 1 h. Following a thorough rinse in PBS containing 0.5% BSA, the sections were then incubated in goat anti-rabbit IgG 10-nm gold complexes (SPI, West Chester, PA) for 1 h and then washed thoroughly in PBS followed by distilled water. The sections were then stabilized in a thin film of methyl cellulose containing 0.2% uranyl acetate before examination in the electron microscope (JEOL JEM 1011, JEOL USA, Peabody, MA). Images were obtained using a 2-K charge-coupled device camera (AMT corp., Danvers, MA). Control images are sections in which primary antibody has been omitted. Generation of morphant zebrafish The morpholino (Gene Tools) was designed against the ATG site of Tmem65 to block translation (5′-GCAACACCGAGCGGAT CAT CAGAGC-3′, with the translation start site underlined). Injection (4 ng) of morpholino at the one-cell stage produced the heart phenotype described. All zebrafish embryo observations were performed on the Leica M205FA fluorescent microscope. The myl7:EGFP twu34 transgenic line, which expresses enhanced green fluorescent protein (eGFP) in myocardial cells, was used in all experiments. Heartbeats were counted manually. To monitor in vivo Ca 2+ transients, the zebrafish were incubated with 0.1% Tricaine (Sigma) and 0.5 μM Fura-2 for 1 h and then washed in water. Calcium transients were acquired using a fluorescence-based image analysis system (Olympus IX81, X-cite 120Q light source from EXFO, Fura 2B filterset from Semrock, using single-band excitation (387 nm) and single-band emission (510 nm), image acquisition with a Rolera MGi plus EM-CCD from Q-Imaging, via the Metamorph v7.6.3. software). Membrane topology Membrane topology of Tmem65 was determined using the MYTH system. To determine protein topography, both N-terminal (TF-Cub-Tmem65) and C-terminal (Tmem65-Cub-TF) ‘bait’ Tmem65 proteins were tested for PPIs in the presence of a non-interacting yeast integral membrane protein Ost1p (ref. 27 ) fused to either NubI (Ost1–NubI) or NubG (Ost1–NubG). The Ost1–NubI control ‘prey’ construct is designed to activate the yeast reporter system, irrespective of a PPI because of the high affinity with which NubI associated with Cub to form active ubiquitin [26] , but only if the Cub domain of the corresponding ‘bait’ protein is localized in the cytosol. Activation of the reporter system was measured as growth on media lacking histidine and adenine in the presence of X-gal. Antibody specificity Specificity of the Tmem65 antibody from Sigma, Abcam and Santa Cruz was probed for by incubating the antibody with Tmem65 overexpressed in HEK293 cells. Western blotting against Tmem65 from adult mouse lysates showed no staining for Tmem65 monomer ( ∼ 22 kDa) or dimer ( ∼ 44 kDa) with the blocked antibody. Dye transfer assay Individual mNCM in a monolayer of plate cells were injected with pyranine with 8-Hydroxypyrene-1,3,6-Trisulfonic Acid, Trisodium Salt dye (Life Technologies) using an in-house developed Robotic Adherent Cell Injection System [68] . Dye transfer measurements were observed 5 min after initial injection [69] . How to cite this article: Sharma, P. et al. Evolutionarily conserved intercalated disc protein Tmem65 regulates cardiac conduction and connexin 43 function. Nat. Commun. 6:8391 doi: 10.1038/ncomms9391 (2015).